Composite fermions and broken symmetries in graphene The electronic properties of graphene are described by a Dirac Hamiltonian with a four-fold symmetry of spin and valley. This symmetry may yield novel fractional quantum Hall (FQH) states at high magnetic field depending on the relative strength of symmetry-breaking interactions. However, observing such states in transport remains challenging in graphene, as they are easily destroyed by disorder. In this work, we observe in the first two Landau levels the two-flux composite-fermion sequences of FQH states between each integer filling factor. In particular, the odd-numerator fractions appear between filling factors 1 and 2, suggesting a broken-valley symmetry, consistent with our observation of a gap at charge neutrality and zero field. Contrary to our expectations, the evolution of gaps in a parallel magnetic field suggests that states in the first Landau level are not spin-polarized even up to very large out-of-plane fields. In a large magnetic field B , the band structure of two-dimensional electrons becomes a discrete set of highly degenerate Landau levels (LLs) [1] , [2] , [3] , [4] . With kinetic energy quenched, the electron interactions determine the ground state of a partially filled LL. This yields new incompressible phases known as fractional quantum Hall (FQH) states [5] , [6] , where the longitudinal resistance ρ xx vanishes exponentially at low temperatures and the transverse resistance ρ xy is quantized as h / νe 2 , where e is the electron charge, h is the Planck’s constant and ν = nh / eB , the number of filled LLs for an electron density n . In GaAs quantum wells, the most robust FQH states are observed when ν = p /(2 kp ±1)=1/3, 2/3, 2/5, 3/5...( k and p integers). This may be understood within the composite fermion (CF) theory, where each electron is imagined to bind an even number 2 k of magnetic flux quanta φ 0 = h / e (refs 7 , 8 , 9 , 10 ). CFs experience an effective residual magnetic field B *= B −2 knφ 0 , and incompressible phases occur when the number of filled CF LLs p = nφ 0 / B * is an integer. In graphene, the ground state in each of these FQH phases is characterized by the two internal degrees of freedom of the Hamiltonian, the spin and the valley isospin, the latter originating from the hexagonal crystal structure of graphene. These grant LLs an approximate SU(4) symmetry [1] , [2] , [3] , [4] broken at high magnetic fields [11] by Zeeman splitting E Z = gμ B B and valley symmetry breaking on order (refs 12 , 13 , 14 ), where a is the graphene lattice constant, l B is the the magnetic length, E c is the the typical energy of Coulomb interactions at a length scale l B and ε is the the dielectric constant. While the nature of the broken-symmetry phases at integer filling factors has been under intense scrutiny [11] , [12] , [13] , [14] , [15] , [16] , [17] , little is known about the impact of symmetry-breaking interactions on FQH states [18] , [19] , [20] , [21] , [22] , [23] , [24] , [25] , [26] . In this work, we present magneto-transport measurements on high-quality graphene devices at magnetic fields up to 45 T and temperatures down to 30 mK. Between each integer filling factor and up to ν =6, we observe sequences of FQH states with unprecedented detail in transport. These follow the two-flux CF sequence δν = p /(2 p ±1), with p ≤5 integer. Several devices are gapped at zero field, as a result of their substrate-induced broken sublattice symmetry. These host FQH states at odd filling factors 5/3 and 7/5, which were absent in devices with a preserved valley symmetry. In addition, we report the first study of the in-plane field dependence of ρ xx at fixed out-of-plane field in the FQH regime of graphene. We observe a pronounced weakening of FQH states in the first LL as the in-plane field is increased, suggesting that they are not yet spin-polarized up to very large field. Characterization at low magnetic field Observation of FQH states requires that disorder-induced Fermi level fluctuations δE F be smaller than FQH energy gaps. To minimize δE F , we place monolayer graphene on an atomically flat flake of hexagonal boron nitride [27] , [28] , which is typically 15–25 nm thick in the seven heterostructures we studied. The carrier density is tuned with a voltage V BG applied to a graphite back gate ( Fig. 1a ), which also acts as a screening layer, recently shown to make the potential landscape in graphene devices cleaner [29] , [30] , [31] . Potential fluctuations should be suppressed on length scales larger than the distance to the back gate, while electron interactions remain on the scale of the magnetic length , less than the distance to the back gate for the relevant magnetic field range. The devices included in this study have field-effect mobilities ranging from 4 × 10 5 to 10 6 cm 2 V −1 s −1 , as extracted from a linear fit to the conductivity σ ( n ) at low density (typically n <2 × 10 11 cm −2 ). This high quality is seen from the longitudinal resistivity ρ xx , plotted in logarithmic scale as a function of the carrier density for Device A, at temperature T =4 K and B =0 T ( Fig. 1b ). ρ xx drops to 20 Ω at n =5 × 10 12 cm −2 , although in this regime the mean free path is limited by boundary scattering [32] and the sheet resistivity is not well defined. The quantum mobility is also estimated from the onset of the ν =2 gaps in ρ xx ( V BG , B ) (ref. 33 ), which for example occurs at 25 mT for Device B ( Fig. 1b , inset), indicating a mobility of at least 4 × 10 5 cm 2 V −1 s −1 . 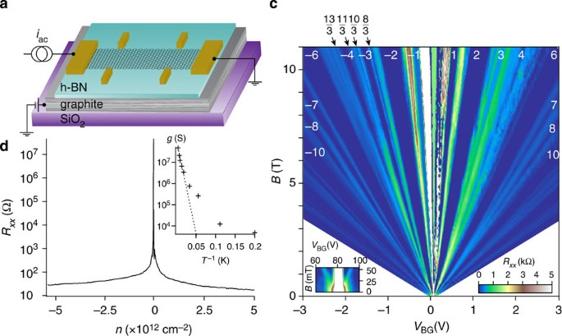Figure 1: Characterization at low field. (a) Schematic of the device, consisting of a graphene/h-BN/graphite stack resting on SiO2.VBGis applied to the graphite back gate to tune the carrier density. (b)ρxx(n) in logarithmic scale, measured atB=0 T andT=4 K. Inset:ρxx(n,B) at very low field and density. (c) Fan diagram ofρxx(n,B) up to 11 T. Figure 1: Characterization at low field. ( a ) Schematic of the device, consisting of a graphene/h-BN/graphite stack resting on SiO 2 . V BG is applied to the graphite back gate to tune the carrier density. ( b ) ρ xx ( n ) in logarithmic scale, measured at B =0 T and T =4 K. Inset: ρ xx ( n , B ) at very low field and density. ( c ) Fan diagram of ρ xx ( n , B ) up to 11 T. Full size image Five of our seven devices are strongly insulating at the charge neutrality point, with the peak resistivities ρ NP exceeding 100 kΩ at 4 K, well above the theoretical limit of πh /4 e 2 ~20 kΩ expected for gapless pristine graphene [34] , [35] , [36] (the last two devices are comparable in quality but with ρ NP <20 kΩ). This phenomenon has only been seen in extremely clean graphene on boron nitride [29] , [30] and has been attributed to sublattice symmetry breaking [29] , [30] , [37] , [38] , [39] . We made no attempt to rotationally align our graphene and BN flakes, suggesting that very close rotational alignment is not required to produce this insulating behaviour (in agreement with ref. 30 , where a graphene flake with misalignment up to 4° on BN still showed activated transport). In only two of our five insulating devices do we see superlattice peaks at attainable densities (5.3 and 6.0 × 10 12 cm −2 , respectively), indicating a rotational misalignment under 1.5° (see Supplementary Note and Fig. 1 ). In our most insulating device (Device A), ρ xx ( V BG ) spans six orders of magnitude up to 20 MΩ at the neutrality point ( Fig. 1b , in log scale). The temperature dependence of its peak resistivity is activated above 20 K ( Fig. 1b ): an Arrhenius fit ρ xx ~exp(−Δ/2 k B T ) yields a gap Δ=350±60 K, similar to that reported recently [30] . As B is increased, vanishing ρ xx indicates quantum Hall phases at integer filling factor (dark blue regions on Fig. 1c ). Broken-symmetry states ν =1 and 3 are visible at B ~1.5 T, and the zero field insulating state continuously undergoes a transition to the ν =0 phase below 1 T (refs 29 , 30 . Remarkably, FQH states at ν =−8/3, −10/3, −11/3 are seen for B as low as 5 T, significantly lower than in refs 40 , 41 , 42 . From now on we focus on FQH states in the hole-doped regime. Contrary to the case of bilayer graphene [43] , the sequence of FQH states in monolayer graphene is electron–hole symmetric, but our data are significantly cleaner on the hole side. We suppress the negative sign of ν when we refer to values of filling factor. FQH effect in the zeroth LL The zeroth LL in monolayer graphene is populated at filling factors | ν |≤2. Between ν =0 and 1, we observe a detailed series of FQH states following the two-flux composite-fermion sequence [44] at ν (or 1− ν )=1/3, 2/5, 3/7, 4/9 ( Fig. 2a ). Corresponding plateaus appear in the transverse conductivity , despite modest mixing between the longitudinal and transverse signals. 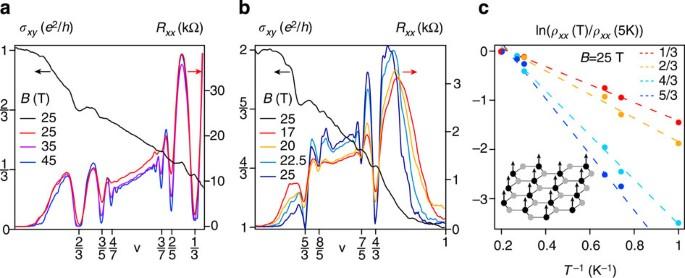Figure 2: FQH effect in the zeroth LL. (a)ρxx(v) betweenv=0 andv=1 at 25 T (red), 35 T (purple) and 45 T (blue). At 45 T, FQH states with denominator 9 are noticeable.σxy(black curve) shows well-defined plateaus at 2/3, 3/5 and 4/7. At lower filling factors, mixing withρxxmakes the plateaus indistinct. (b)ρxx(v) betweenv=1 andv=2 forBranging from 17 to 25 T. FQH states are visible at 5/3 and 7/5, not just even-numerator fractions.σxy(black curve) at 17 T. (c) Arrhenius plots forv=1/3, 2/3, 4/3 and 5/3, showing activated behaviour. Figure 2: FQH effect in the zeroth LL. ( a ) ρ xx ( v ) between v =0 and v =1 at 25 T (red), 35 T (purple) and 45 T (blue). At 45 T, FQH states with denominator 9 are noticeable. σ xy (black curve) shows well-defined plateaus at 2/3, 3/5 and 4/7. At lower filling factors, mixing with ρ xx makes the plateaus indistinct. ( b ) ρ xx ( v ) between v =1 and v =2 for B ranging from 17 to 25 T. FQH states are visible at 5/3 and 7/5, not just even-numerator fractions. σ xy (black curve) at 17 T. ( c ) Arrhenius plots for v =1/3, 2/3, 4/3 and 5/3, showing activated behaviour. Full size image The sequence of FQH states between ν =1 and 2 is more intriguing: the transport and local compressibility measurements [40] , [44] , [45] in graphene both suspended and on boron nitride have lacked incompressible states at odd-numerator fractional filling factors. The associated ground states are believed to be spin-polarized, but susceptible to valley-textured excitations [46] . Unlike more familiar spin skyrmions [47] , spin-polarized valley skyrmions can be spatially extended even at high magnetic fields [46] because they do not involve spin flips. They provide low-lying delocalized excitations and explain the absence of incompressible states at these odd-numerator fractions in refs 40 , 44 . Yet in Fig. 2b , we see minima of ρ xx not only at even-numerator filling factors 4/3 and 8/5 but also at 5/3 and 7/5. These were absent in refs 40 , 44 and suggest that the valley skyrmions are suppressed in our samples. We extract activation gaps from Arrhenius fits to the temperature dependence of ρ xx at 25 T ( Fig. 2c ). Surprisingly, we find Δ 5/3 to be the most robust at 10.4±1.4 K, followed by Δ 4/3 =8.9±0.6 K, Δ 2/3 =4.6±0.3 K and Δ 1/3 =3.5±0.2 K. Theoretical estimates of these gaps are one order of magnitude larger. Δ 4/3 and Δ 2/3 were predicted to be the largest gaps, ranging from 0.08 to 0.11 e 2 /ε l B (or ), for ε=(1+ε BN )/2≈2.5) (refs 21 , 24 ). Theoretical estimates for Δ 1/3 and Δ 5/3 are slightly smaller: 0.03 to 0.1 e 2 /ε l B (or ) (refs 24 , 48 ). The observed gaps are most likely reduced relative to predictions due to disorder, the density at which FQH states occur fluctuating spatially due to remaining charged impurities [44] . This sensitivity to disorder causes FQH gaps to sometimes decrease after successive cool downs and to vary slightly between samples. It is also possible that gaps are reduced as filling factors approach ν =0 due to the competing insulating phase at charge neutrality [40] , [44] . The boron nitride substrate can dramatically affect the band structure of graphene due to the very similar crystal lattices of these two materials [49] . Satellite Dirac peaks emerge at high densities [30] , [50] , [51] and the quantum Hall spectrum changes dramatically, exhibiting a fractal pattern known as the Hofstadter butterfly when l B is comparable to the superlattice moiré cell size [30] , [50] , [51] . We observed superlattice effects in some of our devices at very high densities ( Supplementary Fig. 1 ), but restricted our study to samples and ranges of ( n , B ) where such effects do not impact the quantum Hall spectrum. Even for twist angles up to a few degrees, boron nitride may break the sublattice symmetry [30] , [38] , resulting in a zero-field insulating behaviour at the neutrality point as observed in Fig. 1b [29] , [30] . In the zeroth LL, wavefunctions corresponding to the two valleys are each localized on a different sublattice. Sublattice symmetry breaking should therefore yield valley-polarized ground states, making extended valley skyrmions energetically costly. This is consistent with the observation of FQH states at ν =5/3 (ref. 30 ) and 7/5 in samples that are also gapped at zero field. FQH effect in the first LL FQH states in the first LL of graphene were predicted to be much more robust than in non-relativistic two-dimensional electron gases (2DEGs) [48] , [52] ; yet, only states with denominator 1/3 have been reported in transport and scanning compressibility measurements have not reached sufficient density to probe beyond the zeroth LL. In contrast, we observe a detailed sequence of FQH states in transport, with sharp local minima of ρ xx visible at factors ν + δν , where ν =2, 3, 4 and δν =1/3, 2/3, 2/5, 3/5, 3/7, 4/7... ( Fig. 3a , Device A, T =300 mK). Minima of ρ xx occur at constant filling factors (vertical blue lines) indicating that they are indeed FQH states, some of them emerging at particularly low fields. Between ν =2 and 3, additional FQH states are noticeable at 45 T, such as 17/7, 22/9 and 27/11 ( Fig. 3f ). We do not observe fractions beyond ν =5 and even the integer QH state ν =5 is not always clearly defined, a feature we have observed in several devices and cannot presently explain. 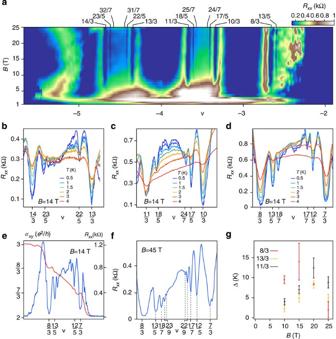Figure 3: FQH Effect in the first LL. (a)ρxx(n,B) fromv=2 tov=5, measured at B=14 T, T=30 mK (Device B). FQH states follow the CF sequencep/(2p±1) between each integer up tov=5. 7/3 is poorly resolved in this device, but this is not a generic feature. No FQH states are seen beyondv=5. (b–d) Temperature dependence of the FQH states in thev=2 to 3,v=3 to 4 andv=4 to 5 sequences (Device A). Temperatures range from 500 mK to 4 K.ρxxexponentially vanishes asTis lowered. Contrary to Device B, the 7/3 state is visible in this device. (e)ρxxandσxyin thev=2 to 3 sequence, measured at B=14 T and T=30 mK (Device A). Plateaus ofσxyare seen at filling factors 7/3, 12/5, 13/5, 8/3. FQH states are observed inρxxatv=17/7 and 18/7 but are not resolved inσxy. (f)ρxxobserved in thev=2 tov=3 sequence (45 T, T=400 mK, Device A). FQH states are observed at denominators up to 11. (g) Field dependence of the activation gaps for Device B atv=8/3 (red), 11/3 (black) and 13/3 (yellow). Error bars correspond to 1-σconfidence interval. Figure 3: FQH Effect in the first LL. ( a ) ρ xx ( n , B ) from v =2 to v =5, measured at B=14 T, T=30 mK (Device B). FQH states follow the CF sequence p /(2 p ±1) between each integer up to v =5. 7/3 is poorly resolved in this device, but this is not a generic feature. No FQH states are seen beyond v =5. ( b – d ) Temperature dependence of the FQH states in the v =2 to 3, v =3 to 4 and v =4 to 5 sequences (Device A). Temperatures range from 500 mK to 4 K. ρ xx exponentially vanishes as T is lowered. Contrary to Device B, the 7/3 state is visible in this device. ( e ) ρ xx and σ xy in the v =2 to 3 sequence, measured at B=14 T and T=30 mK (Device A). Plateaus of σ xy are seen at filling factors 7/3, 12/5, 13/5, 8/3. FQH states are observed in ρ xx at v =17/7 and 18/7 but are not resolved in σ xy . ( f ) ρ xx observed in the v =2 to v =3 sequence (45 T, T=400 mK, Device A). FQH states are observed at denominators up to 11. ( g ) Field dependence of the activation gaps for Device B at v =8/3 (red), 11/3 (black) and 13/3 (yellow). Error bars correspond to 1- σ confidence interval. Full size image As expected, ρ xx minima have a strong temperature dependence, captured at 14 T for a different device (B) in Fig. 3b–d for temperatures between 500 mK and 4 K. For each filling factor, ρ xx ( T ) is fitted to an Arrhenius law ρ xx ( v )~exp(−Δ ν /2 k B T ). At that field, we find Δ 8/3 =5.5±1.5 K and Δ 10/3 =6.3±2.1 K, while Δ 7/3 =5.4±1.4 K, Δ 13/3 =1.2±0.2 K and Δ 14/3 =2.3±0.5 K. The temperature dependence of ρ xx (11/3) is not strong enough to extract a gap value. As expected, FQH states with higher denominator are weaker than denominator-3 states at nearby filling factors, with Δ 12/5 =1.4±0.3 K, Δ 13/5 =2.6±0.8 K and Δ 17/5 =1.8±0.4 K. Probing the nature of the FQH states The extracted gaps are at least one order of magnitude smaller than theoretically predicted, and are likely reduced by disorder. In addition, their perpendicular field ( B ⊥ ) dependence does not follow that of the Coulomb energy at the magnetic length scale . Rather, the field dependence we observe is not monotonic in the first LL, with a noticeable decrease at high fields we did not observe in the zeroth LL (Device A, Fig. 3g ). This could be due to emerging superlattice effects at high field and density, or to approaching FQH phase transitions between different ground states. To probe the spin-polarization of the ground states at each filling factor, we follow the evolution of the gap when the sample is tilted with respect to B , which allows us to change the relative strength of the Zeeman coupling, proportional to the total field B , and Coulomb interactions, controlled by the perpendicular field B ⊥ ( Fig. 4 , inset). In what follows, we call the in-plane field B || , so . Previous graphene transport measurements in the FQH regime required very large B ⊥ , making it challenging to tilt samples with respect to the magnetic field while preserving FQH states. Here the fractions are observed at fields as low as 6 T, so we can measure ρ xx at a fixed B ⊥ =17 T while substantially changing the total field ( Fig. 4 ). In the zeroth LL, the minima of ρ xx at ν =−5/3, −4/3, −2/3, −3/5, −2/5 and −1/3 do not change strength when increasing B || with B ⊥ fixed. This observation is consistent with all ground and low-lying excited states being spin-polarized, in agreement with the theoretical expectations between ν =−2 and −1, where less than a quarter of the zeroth LL is filled and electrons in a FQH state can occupy a single hyperspin state with spins aligned with B (ref. 46 ). Between ν =−1 and 0, however, full spin-polarization would be surprising: electrons should occupy at least two hyperspin states, and based on the zero-field insulating behaviour at the charge neutrality point sublattice symmetry breaking strongly favours valley polarization. This would mean that spins cannot all be aligned with B . The absence of in-plane field dependence for these fractions may mean that the ground state and low-lying excited states have the same (not fully polarized) spin structure, or simply that the Zeeman coupling remains small compared with a particularly large gap associated with the broken-valley symmetry of the zeroth LL, especially in samples such as these, where the sublattice symmetry is broken by the BN substrate. 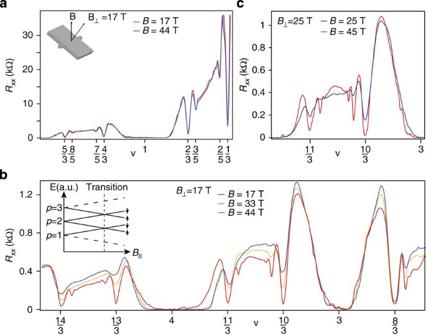Figure 4: In-plane field dependence of the FQH states in the first two LLs of Device B at T=400 mK. (a)ρxx(ν) betweenν=0 andν=2 (B⊥=17 T,B=17 and 44 T). (b)ρxx(ν) betweenν=2 andν=5 (B⊥=17 T,B=17, 33 and 44 T). Inset: schematic of the in-plane field dependence of the CF LL energies at fixedB⊥. (c)ρxx(ν) betweenν=3 andν=4 (B⊥=25 T,B=25 and 45 T). Figure 4: In-plane field dependence of the FQH states in the first two LLs of Device B at T=400 mK. ( a ) ρ xx ( ν ) between ν =0 and ν =2 ( B ⊥ =17 T, B =17 and 44 T). ( b ) ρ xx ( ν ) between ν =2 and ν =5 ( B ⊥ =17 T, B =17, 33 and 44 T). Inset: schematic of the in-plane field dependence of the CF LL energies at fixed B ⊥ . ( c ) ρ xx ( ν ) between ν =3 and ν =4 ( B ⊥ =25 T, B =25 and 45 T). Full size image This behaviour contrasts with our observations in the first LL, where most FQH gaps are seen to decrease with B || ( Fig. 4b and Supplementary Fig. 2 ). Minima at 17/5 and 18/5 disappear, while 10/3 and 11/3 are visibly weakened. Only 8/3 remains robust. We observed the same behaviour in two different samples at perpendicular field up to 25 T ( Supplementary Note 2 ). We would naively expect that such a high field should be strong enough to completely polarize the spin, but gaps weakened by increasing B || suggest instead that the first LL FQH ground states are not yet spin-polarized even at 25 T. Integer quantum Hall gaps follow a similar evolution than the one observed in ref. 12 : at half-filling, the region of vanishing ρ xx widens with B || suggesting a strengthening of Δ 4 , while gaps at quarter-filling Δ 3 and Δ 5 remain the same. This was attributed in ref. 12 to a spin-polarized ground-state at ν =4 with low-lying excitations involving spin flips, while ground states at quarter-filling have valley-textured excitations. The spin-polarization of the ground state at a given filling factor depends on the competition between electron interactions and the Zeeman splitting. Neglecting spin, FQH gaps between two successive integer filling factors are expected to scale like Coulomb interactions, with Δ ν ∝ |1−2 δν | e 2 /ε l B , where δν = p /(2 p +1). The prefactor |1−2 δν | stems from the effective field B *= B ⊥ |1−2 δν | experienced by CFs, which vanishes when approaching half-filling. This explains the decreasing gaps for FQH states with high index p , a well-documented fact in GaAs-based 2DEGs (refs 53 , 54 ). For CFs with a spin, the spin-polarization of the ground state at a given filling factor depends on the competition between electron interactions and the Zeeman splitting [55] , [56] : Zeeman splitting of the two consecutive CF LLs should produce a LL crossing when gμB equals the Coulomb contribution to the gap stated above, which only scales like . Below the transition, activation gaps should decrease linearly with an in-plane field, which could explain our observations in the first LL. Such crossings and associated transitions of ground states have been observed in transport in GaAs-based 2DEGs (ref. 53 ), and more recently in the zeroth LL of graphene using compressibility measurements [45] . How should field scales for these transitions differ between GaAs and graphene? The dielectric constant is five times lower in graphene on BN than in GaAs, so at a given field electron interactions are stronger in graphene. Yet, Zeeman splitting is also much larger in graphene, with g ≥2 compared with g ≈0.4 in GaAs, and it is therefore unclear why the field required to observe transitions to spin-polarized states should be larger in graphene. However, for a given ratio e 2 /ε l B , FQH gaps in the first LL of graphene were predicted to be significantly stronger than gaps in both non-relativistic 2DEGs [48] , [52] and graphene’s zeroth LL, a result of the peculiar form factor of relativistic electron in n ≠0 LLs. We could not quantitatively compare gaps between zeroth and first LLs at the same field in our devices ( Supplementary Note 3 ). However, at low field ( B ≤14 T), several devices showed better developed FQH states in the first LL ( Supplementary Fig. 3 ), in qualitative agreement with theoretical expectations [48] , [52] . This could explain the need for larger Zeeman splitting to overcome interaction-induced gaps in the first LL and induce phase transitions to spin-polarized states, but would not explain what is special about ν =8/3, the only fractional state in the first LL which is not weakened by an in-plane field at B ⊥ =17 T. Fabrication The graphene/h-BN/graphite structure is fabricated using the transfer method described infit [29] , [57] . Few-layer graphite is exfoliated on SiO 2 . Graphene and h-BN flakes are separately exfoliated on a polymer stack of polymethyl-methacrylate (400 nm) atop polyvinyl alcohol (60 nm). We transfer h-BN first, then graphene, on top of the graphite flake. For each transfer, the polyvinyl alcohol is dissolved in deionized water, the PMMA membrane lifts-off, is transferred on a glass slide, heated at 110 °C and aligned on top of the target with a micromanipulator arm. After each transfer, samples are annealed in flowing argon and oxygen (500 and 50 s.c.c.m. respectively) in a 1" tube furnace at 500 °C to remove organic contamination [58] . E-beam lithography is combined with oxygen plasma etching to define the graphene flake geometry, and with thermal evaporation to deposit Cr/Au contacts (1 nm/100 nm). Measurement The devices were measured in a 3 He cryostat and a dilution fridge in a current-biased lock-in setup, with an ac excitation current of 20 nA at 13 Hz. Measurements at fields higher than 14 T were performed at the National High Magnetic Field Laboratory in Tallahassee. How to cite this article : Amet, F. et al . Composite fermions and broken symmetries in graphene. Nat. Commun. 6:5838 doi: 10.1038/ncomms6838 (2015).